Subnuclear gene positioning through lamina association affects copper tolerance The nuclear lamina plays an important role in the regulation of chromatin organization and gene positioning in animals. CROWDED NUCLEI (CRWN) is a strong candidate for the plant nuclear lamina protein in Arabidopsis thaliana but its biological function was largely unknown. Here, we show that CRWNs localize at the nuclear lamina and build the meshwork structure. Fluorescence in situ hybridization and RNA-seq analyses revealed that CRWNs regulate chromatin distribution and gene expression. More than 2000 differentially expressed genes were identified in the crwn1crwn4 double mutant. Copper-associated ( CA ) genes that form a gene cluster on chromosome 5 were among the downregulated genes in the double mutant exhibiting low tolerance to excess copper. Our analyses showed this low tolerance to copper was associated with the suppression of CA gene expression and that CRWN1 interacts with the CA gene locus, enabling the locus to localize at the nuclear lamina under excess copper conditions. Chromatin does not drift in the nucleoplasm but instead associates with inner nuclear membranes, the nuclear lamina, nuclear pores, the nucleolus, and nuclear bodies, all of which are components responsible for the non-random spatial positioning of genomic loci [1] , [2] . Several studies have suggested that gene positioning in the three-dimensional subnuclear space affects transcriptional activity [3] . In budding yeast, several genes are located at the nuclear periphery when they are activated [4] , [5] , [6] , [7] . In many types of mammalian cells, inactivated genes are positioned at the nuclear periphery, while activated genes are localized around the center of the nucleoplasm [8] . However, the effects of gene positioning on transcription in plants are unknown. As the location of a gene at the nuclear periphery can affect its expression, the nuclear lamina plays important roles as a platform for gene localization and/or expression. The nuclear lamina, a meshwork structure beneath the inner nuclear membrane, has been observed in animal and plant cells [9] , [10] . In metazoans, the nuclear lamina is mainly composed of lamins, which interact with each other via their central rod domain containing four coiled-coil regions to form intermediate filaments and a meshwork structure that mechanically supports the nuclear membrane [11] , [12] . Lamins can directly and/or indirectly bind to chromatin to control the distribution and positioning of chromatin and gene activity. Nuclear lamina-associated domains (LADs) have been identified and mapped in animal cells by chromatin immunoprecipitation (ChIP) and DNA adenine methyltransferase identification (Dam-ID) methods. The LADs include low-expression genes, gene-free genomic regions, and repeat sequences such as pericentromeres, and are enriched in histone modifications for heterochromatin [13] . Although lamin homologs have not been found in plant genomes, the meshwork structure has been observed in the nuclear lamina by electron microscopy, which implies that unidentified proteins make up the nuclear lamina structure [10] , [14] . The crowded nuclei (CRWN) proteins are strong candidates for functional lamin-like proteins. CRWNs were first identified as nuclear matrix constituent proteins (NMCPs) from carrot and are widely conserved in land plants [15] . Like lamins, CRWNs contain a long coiled-coil region at their N-terminal. Arabidopsis thaliana harbors four CRWN homologs that are phylogenetically separated into two groups: the NMCP1 group, including CRWN1, CRWN2, and CRWN3; and the NMCP2 group including CRWN4 [16] , [17] . In previous studies, CRWNs were detected in the nuclear lamina fraction and localized at the nuclear periphery [18] . Single or double crwn mutants have small and abnormally shaped nuclei [16] , [18] . Double mutants and some triple mutants have a dwarf phenotype, and some triple and quadruple mutants are lethal [19] . CRWN1 and CRWN3 play roles in seed dormancy by inhibiting the degradation of ABI5 [20] . CRWNs are also involved in resistance against virulent bacterial pathogens [21] . CRWN1 is degraded in a proteasome-mediated manner in response to pathogens, resulting in activation of the plant immune response gene pathogenesis-related protein 1 (PR1). Here, we report that CRWNs form the meshwork structure at the nuclear lamina. We demonstrate that the upregulation of copper-associated genes is required for copper tolerance and is inhibited in crwn1crwn4 mutants with low copper tolerance. The gene locus interacts with CRWN1 and is anchored to the nuclear periphery, which activates gene expression, only under excess copper conditions. CRWNs specifically localize and build a meshwork structure at the nuclear periphery In contrast to previous studies in which CRWN1–4 proteins were expressed under the control of a strong 35S promoter, we here wanted to test the expression and localization patterns upon expression under the control of the native promoter. Towards this goal, we prepared pCRWN ::CRWN-GUS in the wild type (WT) and pCRWN ::CRWN-EYFP and -sGFP in each crwn mutant (Fig. 1a, b ). EYFP(S65G/V68U/S72A/T203Y) and sGFP(S65T) are variants of the green fluorescent protein [22] , [23] . CRWN-GUS, -EYFP, and -sGFP were driven by the native promoter (defined as the 2-kbp sequence upstream from the start codon). Although we constructed pCRWN4 ::CRWN4-GUS in WT, we did not detect any signals (Supplementary Fig. 1 ). Fig. 1: CRWN expression and localization patterns in Arabidopsis thaliana . a β-Glucuronidase (GUS) signals in young first leaves (8-day-old plant), adult first leaves (14-day-old plant), and primary roots of pCRWN1 ::CRWN1-GUS, pCRWN2 ::CRWN2-GUS, and pCRWN3 ::CRWN3-GUS. Scale bars = 200 µm (top), 1 mm (middle), and 100 µm (bottom). b Confocal fluorescence images of cotyledons and roots showing pCRWN1 ::CRWN1-EYFP in crwn1 , pCRWN2 ::CRWN2-EYFP in crwn2 , and pCRWN3 ::CRWN3-sGFP in crwn3 . EYFP and sGFP signals are green and propidium iodide signals are magenta. Scale bars = 10 µm (top and middle) and 50 µm (bottom). c Transmission electron micrograph of the nucleus in a root meristematic cell. Lower panel shows a magnified image of the broken square in the upper panel. White arrowheads mark gold particle signals. Dotted and broken lines indicate outer and inner nuclear membranes, respectively. Red, orange, and blue areas indicate the nuclear lamina, internal, and external areas, respectively. Scale bars = 200 nm. d Number of gold particles in each area. Data are mean ± SEM. Significance was determined using unpaired two-sided t -test ( n = 5 individual nucleus). Each data point represents a cross mark. e Immunofluorescence images of nuclear surface and nuclear interior. Immunostaining signals are green and DAPI signals are magenta in the merged panel. Scale bar = 5 µm. f Confocal fluorescence images of root epidermal cells in the elongation zone. Scale bar = 5 µm. g STED images of nuclei isolated from 7-day-old seedlings. Lower panels are magnified images of the area indicated by the small square in the upper panels. Scale bars = 5 µm (top) and 1 µm (bottom). Full size image CRWN1–3 showed similar expression and localization patterns (Fig. 1a , b). CRWN1–3 were strongly expressed in the root apical meristem and young leaves but rarely expressed in mature leaves (Fig. 1a ). CRWN1–3 were specifically localized at the periphery in both spherical nuclei and elongated nuclei (Fig. 1b ). To reveal whether CRWNs localized at the nuclear lamina area, pCRWN1 ::CRWN1-EYFP in crwn1 was observed by immunoelectron microscopy using an anti-GFP antibody and a gold-conjugated secondary antibody (Fig. 1c ). The majority of the CRWN1 signals appeared to be observed in the nuclear lamina (Fig. 1c ). To quantify the signals, the nucleus was classified into three areas: the nuclear lamina, internal, and external area. The nuclear lamina area and the external area were the parts within 100 nm of the inner and outer nuclear membranes, respectively. The internal area was the inner region further inside from the nuclear lamina area. Gold particles were more abundant at the nuclear lamina area than at other areas, indicating that CRWN1 specifically localized at the nuclear periphery, suggesting that it could be a major constituent of the plant nuclear lamina (Fig. 1d ). Next, to investigate the distribution of CRWN1 at the nuclear lamina, pCRWN1 ::CRWN1-EYFP was visualized in isolated nuclei by immunofluorescence staining using an anti-GFP antibody. CRWN1 showed the meshwork pattern at the nuclear periphery (Fig. 1e ). In live imaging analysis, pCRWN1 ::CRWN1-EYFP also formed a meshwork pattern at the nuclear periphery in a root epidermal cell (Fig. 1f ). Furthermore, detailed distribution patterns of CRWN1–3 were observed by stimulated emission depletion (STED) microscopy, which is one of the super-resolution microscopies and provides sub-diffraction-limit imaging by using a second laser negating the emission from fluorophores located away from the centre of excitation. CRWN1–3 exhibited similar continuous structures (Fig. 1g ). These results suggested that CRWN1–3 proteins built the meshwork structure at the plant nuclear lamina area. To determine whether CRWNs interact with each other, which is probably required for construction of the meshwork structure, protein–protein interactions were analyzed by co-immunoprecipitation (Co-IP) assay and yeast two-hybrid assay (Y2H). Both assays indicated that CRWN1, CRWN2, and CRWN3 interacted with each other, and that CRWN1 also interacted with CRWN4 (Fig. 2a, b ). However, CRWN4 could not interact with CRWN2 or CRWN3. The homomeric interaction of CRWN3 was detected by Co-IP but not by Y2H and that of CRWN4 was detected by Y2H but not by Co-IP, suggesting that the CRWN3 interaction negatively affected the reporter gene expression in yeast and the CRWN4 interaction was too weak to be detected by Co-IP. These protein interaction assays demonstrated that all CRWNs could form homo- and/or hetero-oligomers for construction of the meshwork structure. Fig. 2: Interactions among CRWNs. a Analysis of the interactions among CRWNs in Nicotiana benthamiana leaves detected by co-immunoprecipitation assay. Data are from single representative experiments that were reproduced twice. b Analysis of the CRWN interactions by yeast two-hybrid assay. Growth tests of yeast expressing CRWNs on agar plates lacking leucine, tryptophan, and histidine (top), or leucine and tryptophan (bottom). Empty vectors of bait (BK) and prey (AD) served as negative controls. Full size image CRWNs regulate chromatin distribution and gene expression To explore the function of CRWNs in chromatin organization, we investigated the chromatin distribution in crwn single and double mutants by fluorescence in situ hybridization (FISH). The number of signals derived from 180-bp pericentromeric sequences was around 10 in WT nuclei, but significantly lower in nuclei of crwn1 , crwn4 , crwn1crwn2 , and crwn1crwn4 , suggesting that CRWNs are involved in the maintenance of chromatin structure and distribution (Supplementary Fig. 2a ). Instead of a reduction of the number of signals, the size and intensity of a signal were increased in the crwn1crwn4 (Supplementary Fig. 2b, c ), suggesting that pericentromeric regions were not lost but aggregated with each other. Next, the RNA-seq analysis of 2-week-old WT and crwn1crwn4 was performed to determine whether the gene expression pattern was also affected by the defect of CRWN1 and CRWN4. Gene expression data were normalized and compared using TCC in the R software package to identify differentially expressed genes (DEGs) between WT and crwn1crwn4 . The DEGs were defined as those with transcript levels greater than 1.5-fold or reduced to less than 0.667-fold and a false-discovery rate (FDR) of less than 0.05. We identified 2122 DEGs (991 upregulated genes and 1131 downregulated genes in crwn1crwn4 vs . WT) (Fig. 3a, b ). The Gene Ontology analysis revealed that, among both up- and downregulated genes, there was the enrichment of biotic and abiotic stress-responsive genes (Fig. 3c ), suggesting that CRWN1 and CRWN4 mainly regulate stress response pathways. Fig. 3: CRWNs affect gene expression pattern. a Scatter plots of RNA-seq data comparing mRNA abundance between WT and crwn1crwn4 . Red marks denote mRNAs upregulated more than 1.5-fold (FDR < 0.05); blue marks denote those downregulated to <0.667-fold (FDR < 0.05); gray marks denote other mRNAs. b Pie chart of differentially expressed genes (DEGs). c Enrichment analysis of GO terms for upregulated genes (top) and downregulated genes (bottom). GO analysis according to biological process. Full size image CRWN1 and CRWN4 regulate transcript levels of copper-associated genes Three copper-associated ( CA ) genes, belonging to the family encoding heavy metal-associated proteins in plants, were among the downregulated DEGs in crwn1crwn4 . Heavy metal-associated domains are conserved among the family members and are involved in the chelating of metal ions in the cytoplasm [24] . The 11 CA genes ( CA1–11 ) including the three genes mentioned above are tandemly localized on the long arm of chromosome 5 (Fig. 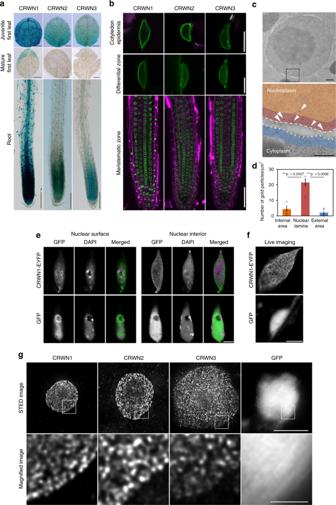Fig. 1: CRWN expression and localization patterns inArabidopsis thaliana. aβ-Glucuronidase (GUS) signals in young first leaves (8-day-old plant), adult first leaves (14-day-old plant), and primary roots ofpCRWN1::CRWN1-GUS,pCRWN2::CRWN2-GUS, andpCRWN3::CRWN3-GUS. Scale bars = 200 µm (top), 1 mm (middle), and 100 µm (bottom).bConfocal fluorescence images of cotyledons and roots showingpCRWN1::CRWN1-EYFP incrwn1,pCRWN2::CRWN2-EYFP incrwn2, andpCRWN3::CRWN3-sGFP incrwn3. EYFP and sGFP signals are green and propidium iodide signals are magenta. Scale bars = 10 µm (top and middle) and 50 µm (bottom).cTransmission electron micrograph of the nucleus in a root meristematic cell. Lower panel shows a magnified image of the broken square in the upper panel. White arrowheads mark gold particle signals. Dotted and broken lines indicate outer and inner nuclear membranes, respectively. Red, orange, and blue areas indicate the nuclear lamina, internal, and external areas, respectively. Scale bars = 200 nm.dNumber of gold particles in each area. Data are mean ± SEM. Significance was determined using unpaired two-sidedt-test (n= 5 individual nucleus). Each data point represents a cross mark.eImmunofluorescence images of nuclear surface and nuclear interior. Immunostaining signals are green and DAPI signals are magenta in the merged panel. Scale bar = 5 µm.fConfocal fluorescence images of root epidermal cells in the elongation zone. Scale bar = 5 µm.gSTED images of nuclei isolated from 7-day-old seedlings. Lower panels are magnified images of the area indicated by the small square in the upper panels. Scale bars = 5 µm (top) and 1 µm (bottom). 4a and Supplementary Table 1 ). Quantitative RT-PCR (qRT-PCR) analyses of 2-week-old plants revealed that half of the genes in this cluster ( CA5 and CA7–10 ) were downregulated in crwn1crwn4 compared with the levels in WT (Fig. 4b ). Interestingly, the expression levels of CA5–10 genes were unchanged in crwn2crwn3 , exhibiting an almost normal chromatin distribution pattern (Fig. 3a and Supplementary Fig. 3 ). These results suggested that CRWN1 and CRWN4 but not CRWN2 and CRWN3 transcriptionally regulate CA genes. Fig. 4: CRWNs elevate expression of CA genes. a Schematic figure of the CA gene locus on chromosome 5. Downregulated genes identified by qRT-PCR are shown in blue and other CA genes are shown in gray. b qRT-PCR analysis of CA genes in 2-week-old WT and crwn1crwn4 plants. Data were normalized to EF1α mRNA levels and are expressed as mean ± SEM relative to the WT value (defined as 1). Significance was determined using unpaired two-sided t -test ( n = 5 individual experiments). Each data point represents a cross mark. c WT, crwn1crwn4 , and crwn2crwn3 grown under normal and excess copper conditions for 2 weeks. d Fresh weight of 2-week-old WT, crwn1crwn4 , and crwn2crwn3 grown under normal ( n = 6 individual experiments) and excess copper conditions ( n = 8 individual experiments). Fresh weights of crwn1crwn4 and crwn2crwn3 were normalized against that of WT to calculate relative fresh weight and are expressed as mean ± SEM. Significance was determined using unpaired two-sided t -test. Each data point represents a cross mark. e qRT-PCR analysis of CA gene transcript levels in 4-, 6-, and 9-day-old WT and crwn1crwn4 under normal and excess copper conditions. Data were normalized to EF1α mRNA levels and are expressed as mean ± SEM relative to the value of 4-day-old WT under normal condition (defined as 1). Significance was determined using unpaired two-sided t -test ( n ≥ 3 individual experiments). f Fresh weight of 2-week-old WT, crwn1crwn4 , and crwn1crwn4 expressing CRWN1-EYFP and CA genes under normal and excess copper conditions. Fresh weights of crwn1crwn4 and crwn1crwn4 expressing CRWN1-EYFP and CA genes were normalized against that of WT to calculate relative fresh weight and are expressed as mean ± SEM. Significance was determined using unpaired two-sided t -test (vs crwn1crwn4 ; n ≥ 3 individual experiments). Each data point represents a cross mark. Full size image CRWNs contribute to copper tolerance by upregulating CA genes Although the function of CA genes has not been revealed, they all contain a heavy metal-associated domain [24] . Thus, we investigated the copper tolerance of crwn mutants. The fresh weight of 2-week-old plants of WT, crwn1crwn4 , and crwn2crwn3 was measured under normal (0.05 µM Cu) and excess copper conditions (50 µM Cu). The fresh weight of crwn1crwn4 was approximately 70% of that of WT under normal conditions, but significantly reduced to approximately 40% of that of WT under excess copper conditions (Fig. 4c, d ). Thus, crwn1crwn4 was hypersensitive to excess copper. In contrast, the fresh weight of crwn2crwn3 under both conditions was similar to that of WT (Fig. 4c, d ). As 2-week-old plants of crwn1crwn4 showed weak tolerance to excess copper, we investigated the transcript levels of CA genes at the early stage (4-, 6-, and 9-day-old seedlings) under both normal and excess copper conditions by qRT-PCR. The transcript levels of CA6–10 were increased in response to excess copper in WT at day 9 (Fig. 4e ). However, the transcript levels of CA7, CA8 , and CA10 were lower in crwn1crwn4 than in WT under excess copper conditions at day 9 (Fig. 4e ). The transcript level of copper/zinc superoxide dismutase (CSD) as a positive control was dramatically elevated by excess copper in WT as well as in crwn1crwn4 (Supplementary Fig. 4 ). To clarify whether low expression of CA genes caused the weak copper tolerance of crwn1crwn4 , we generated transformants overexpressing CA genes in crwn1crwn4 . Almost all of the transgenic plants significantly overexpressed the transgenes compared with the level in the WT (Supplementary Fig. 5). Two individual lines of p35S :: CA10 showed similar expression levels to that of WT but significantly increased levels compared with that of the parental line crwn1crwn4 . The fresh weight of pCRWN1 ::CRWN1-EYFP in crwn1crwn4 (positive control) was significantly greater than that of crwn1crwn4 under both normal and excess copper conditions, suggesting that the cause of the dwarf phenotype was knockout of CRWN s and that CRWN1-EYFP could complement this phenotype (Fig. 4f ). The fresh weights of crwn1crwn4 expressing CA5–7 were similar to that of crwn1crwn4 under both conditions. In contrast, the fresh weights of crwn1crwn4 expressing CA8–10 were significantly greater than that of crwn1crwn4 only under excess copper conditions, except for p35S :: CA10 #6 (Fig. 4f ). These results strongly suggested that the low transcript levels of CA8, CA9 , and CA10 resulted in the weak copper tolerance of crwn1crwn4 . CRWNs alter the position of CA genes in the nucleus We formulated a hypothesis to explain how the nuclear lamina proteins regulate the expression of CA genes. The hypothesis was that the CRWNs change the spatial arrangement of the CA genes in the nucleus through interacting with them, which affects their transcriptional activity. To test this hypothesis, we investigated the interaction between CRWNs and CA genes. Chromatin immunoprecipitation (ChIP) assays using CRWN1-EYFP and anti-GFP antibody failed to identify CRWN1-binding sites. Therefore, we used chromatin integration labeling (ChIL) assay [25] , which is based on an antibody reaction like ChIP but does not require immunoprecipitation. First, we prepared pCRWN1 ::CRWN1-EYFP in crwn1 and p35S ::GFP in WT for the ChIL assay. CRWN1-EYFP and CRWN1-binding DNA were cross-linked with formaldehyde and then primary and secondary antibody reactions were performed to label the CRWN1 (Fig. 5a ). The secondary antibody was conjugated with oligo DNA fragments containing the T7 promoter and Tn5 transposase target sequences. After integration between CRWN1-binding DNA and oligo DNA fragments, RNAs were synthesized from CRWN1-binding DNA by T7 RNA polymerase in vitro. Complementary DNA (cDNA) libraries were constructed from purified RNAs. First, we confirmed that CRWN1-binding sites can be detected by ChIL assay. The possible CRWN1-binding sites were detected by qPCR using the primer pairs designed from sequences within the PR1 promoter and pericentromeric region because it was suggested that a protein complex of CRWN1 and NLT9, which is a gene involved in immune responses, bound to the PR1 promoter under normal conditions [21] and CRWN1 interacted with centromeric and pericentromeric regions [26] . The PR1 promoter and pericentromeric region were significantly accumulated in CRWN1 ChILed DNA compared with the level in the control, which suggested that the ChIL assay can reveal the CRWN1-binding sites (Supplementary Fig. 6 ). CRWN1-binding sequences were detected by qPCR using 12 primer pairs designed from sequences within the cluster of CA genes (Fig. 5b ). The values obtained in the CRWN1 ChIL-qPCR were normalized to those obtained in the GFP ChIL-qPCR. In the CRWN1 ChIL-qPCR analysis, specific enrichment of the CA gene locus was not detected under normal conditions, but the position 1 (p1), p3, p5, and p8 fragments were significantly enriched only under excess copper conditions (Fig. 5b ). This suggested that the CA gene locus interacted with CRWN1 in a manner dependent on the amount of copper. Fig. 5: CRWNs regulate the position of the CA gene locus depending on copper concentration. a Outline of chromatin integration labeling (ChIL) method. b ChIL-qPCR analyses using 12 primer pairs described as p1 to p12. Top image indicates the position of primer pairs at the CA gene locus. Data were normalized to ChILed DNA levels in GFP control and are expressed as mean ± SEM. Significance was determined using unpaired two-sided t -test ( n ≥ 4 individual experiments). Each data point represents a cross mark. c , d ChIP assay for histone H3 ( c ) and H4 acetylation ( d ) in the CA gene locus under normal and excess copper conditions. Data are expressed as mean ± SEM. Significance was determined using unpaired two-sided t -test ( n = 3 individual experiments). Each data point represents a cross mark. e Visualization of the CA gene locus in the nucleus by padlock FISH. In the merged panel, FISH signals are red and DAPI signals are cyan. Scale bar = 5 µm. Data are from single representative experiments that were reproduced three times. f The distance between the CA gene locus and the nuclear edge was measured. The red bars in the histogram represent the nuclear periphery including the region 0.0 to 0.2 μm from the nuclear edge. The average percentage of the CA gene locus within the nuclear periphery with SEM from three independent replicates is shown. “ n ” represents the total number of FISH signals analyzed from all replicates. The CA gene locus distribution data under normal conditions were compared with those under excess copper conditions in WT and crwn1crwn4 . Significance was determined using unpaired two-sided t -test. Full size image Next, we performed ChIP assay for histone H3, H4 acetylation (H4ac) as an epigenetic mark of transcriptionally active chromatin, and H3 lysine 27 trimethylation (H3K27me3) as a mark of inactive chromatin to evaluate the chromatin status on the CA gene locus. Under normal conditions, no differences were detected between WT and crwn1crwn4 ; however, under excess copper conditions, the amount of H3 was significantly reduced on p1, p5 and p7, and H4ac was increased on p2 and p3 in WT compared with the levels in crwn1crwn4 (Fig. 5c, d ). This suggested that histones were removed and chromatin was loosened in the CA locus to activate gene expression in response to the excess copper. H3K27me3 showed a similar pattern between WT and crwn1crwn4 (Supplementary Fig. 7 ). Finally, we determined whether the interaction between CRWNs and the CA gene occurred in the nuclear lamina. First, we checked the localization of CRWN1 under normal and excess copper conditions (Supplementary Fig. 8 ). 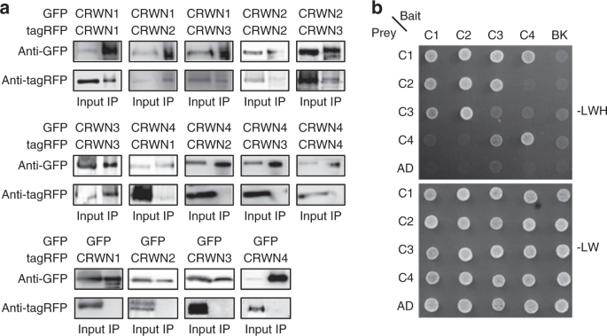Fig. 2: Interactions among CRWNs. aAnalysis of the interactions among CRWNs inNicotiana benthamianaleaves detected by co-immunoprecipitation assay. Data are from single representative experiments that were reproduced twice.bAnalysis of the CRWN interactions by yeast two-hybrid assay. Growth tests of yeast expressing CRWNs on agar plates lacking leucine, tryptophan, and histidine (top), or leucine and tryptophan (bottom). Empty vectors of bait (BK) and prey (AD) served as negative controls. CRWN1 was localized at the nuclear periphery under both conditions. We also checked the position of the CA gene locus by padlock FISH, which can visualize not only repetitive sequences but also a single gene locus in the nucleus [27] (Fig. 5e and Supplementary Fig. 9a ). We defined the nuclear periphery as the area 0.2 µm or closer to the nuclear edge, in accordance with a previously described method [27] . The percentage of the CA gene locus localized at the nuclear periphery was significantly increased from 22 ± 6% under normal conditions to 43 ± 5% under excess copper conditions in WT (Fig. 5d , e). Interestingly, the percentages of the CA gene locus at the nuclear periphery were similar under the two conditions in crwn1crwn4 . In other words, the CA gene positioning was not altered in response to copper stress in crwn1crwn4 . These results suggested that CRWNs mediate the change in CA gene positioning through interacting with the gene locus. Here, we show that CRWNs localize at the nuclear lamina and form interactions that build the meshwork structure. The CA gene locus, at which CA genes are tandemly localized, interacts with CRWN1 and shifts to the nuclear periphery when the genes are activated under excess copper conditions, indicating that CRWN-dependent gene positioning is associated with CA gene activity and copper tolerance. When excess copper ions enter the cell, they should be immediately chelated and discharged by cytoplasmic proteins or chemicals to protect the cytoplasm from copper toxicity. CA genes might be involved in the chelating of copper ions in a manner similar to that for other heavy metal-associated proteins [24] . In fact, excess copper ions activate the expression of CA genes (Fig. 4b, c ). Clustered genes like the CA genes are well known as operons in prokaryotes. The genes clustered together in an operon are co-regulated by a single promoter and operator and are co-transcribed into a single mRNA, which leads to the production of a polycistronic mRNA [28] . Operons have also been discovered in eukaryotes such as Caenorhabditis elegans [29] . Prokaryotic operons form a polycistronic mRNA, whereas C. elegans operons form a polycistronic pre-mRNA, which is subsequently divided into monocistronic mRNAs. Both operon types are transcribed from single promoters and produce polycistronic pre-mRNA or mature mRNA, resulting in the synchronized expression of the clustered genes. Operon-like gene clusters have also been reported in A. thaliana [30] , [31] , [32] . The genes in a cluster are coordinately expressed, although they each have a promoter and are not co-transcribed into a single pre-mRNA and mature mRNA; hence, the regulatory mechanisms of the coordinated expression were not revealed. In this study, the clustered CA genes were transcriptionally co-regulated in response to excess copper. We propose that nuclear positioning of the CA genes impacts on their transcriptional activity. The positioning of genes is positively regulated and affects their expression levels during cell differentiation, maturation, and tissue development in animals [33] , [34] , [35] . Generally, heterochromatin is mainly localized at the nuclear periphery and euchromatin is in the nucleoplasm in animals. Similar tendencies were observed in plants, according to a study on the genomic regions bound to the nucleoporin NUP1, which is a subunit of the nuclear pore complex (NPC) [36] . A ChIP-seq analysis of NUP1 revealed that its binding regions are enriched in silenced genes, transposable elements, and heterochromatin. In addition, recently, CRWN1-binding regions that are similar to NUP1-binding regions were also reported [26] . Silenced biosynthetic gene clusters approach the nuclear periphery, while activated clusters relocate away from it [37] . Other studies found that chromocenters are specifically localized at the nuclear periphery [38] . These results suggest that the nuclear periphery was occupied by heterochromatic and inactive regions in plants. However, some reports suggest that the nuclear periphery can activate gene expression. The nucleoporin Seh1 conjugated with LacI and YFP (She1–LacI–YFP) and LacO fused to the luciferase reporter gene (LacO:Luc) were co-expressed in A. thaliana to investigate the effect of the positioning of genes on their expression [39] . She1–LacI–YFP was localized at the nuclear periphery. Through the strong interaction between LacI protein and LacO DNA sequence, LacO:Luc was probably located at the nuclear periphery and the expression level of Luc was elevated compared with that of the control plants expressing only LacO:Luc. A report has been published on gene repositioning in plants focusing on the chlorophyll a/b-binding protein (CAB) gene locus, where three CAB genes are tandemly located [27] . The locus of the CAB genes, which are involved in de-etiolation, moves from the nucleoplasm to the nuclear periphery in response to red and far-red light. The repositioning of this locus induces a dramatic activation of CAB genes. The repositioning of this locus does not occur in phytochrome signaling mutants, suggesting that light-dependent repositioning of the CAB gene locus is mediated by the phytochrome signaling pathway. However, the molecular mechanism of tethering to the nuclear periphery has not been elucidated. The activation of CA genes at the nuclear periphery is consistent with a previous report describing luciferase gene and CAB gene activation at the nuclear periphery. These results suggest that the nuclear periphery in plants could be divided into gene-activating and -suppressing regions. The findings from the present study showed that the expression of the CA7 , CA8 , and CA10 genes was upregulated whereas CRWN1 interacted with CA3 , CA5 , and CA8 in response to excess copper in 9-day-old plants. Under excess copper conditions, the levels of histone H3 in CA3 , CA5 , and upstream of CA8 were higher and that of H4ac in CA5 was lower in crwn1crwn4 than in WT (Fig. 5c, d ). CRWN1-binding sites and the site where histone was acetylated and removed overlapped, suggesting that the acetylation and removal of histones in the gene locus may be required for the interaction between the CA gene locus and CRWN1, rather than activation of the CA genes. Our study indicated that CRWNs could tether the CA genes to the nuclear periphery; however, no activated genes were present in the CRWN1-binding site and it has not been reported that CRWNs directly regulate gene expression. Other proteins are probably involved in regulating the transcriptional activity of the CA genes. In a previous study, the gene clusters involved in stamen development were identified in A. thaliana [40] . The clustered gene expression was consistently downregulated in the hta9hta11 double mutant exhibiting mutations in two H2A.Z genes, but not in other mutants including haf1 (histone acetyltransferase), atx1 (H3K4 methyltransferase), and ref6 (H3K27 demethylase). In the case of the CA genes, histone variants may be involved in the regulation of gene activation. It was also reported that transcription factors are closely related to gene regulation in a manner dependent on gene positioning in yeast and animal cells [2] . The putative transcription factor bZIP18 was shown to interact with plant-specific nuclear envelope-associated proteins (NEAPs) in A. thaliana [41] . SUNs also bind to both NEAPs and CRWNs, suggesting that CRWNs indirectly interact with bZIP18 [42] . Therefore, bZIP18 may regulate transcriptional activity at the nuclear periphery. Transcriptome analysis of crwn1crwn4 revealed that CRWNs play roles in gene regulation. Among the DEGs, similar numbers of up- and downregulated genes were identified, suggesting that CRWNs are involved in both enhancing and silencing genetic pathways. For example, the CA genes were inhibited in crwn1crwn4 in our study, whereas the expression of a gene involved in immune responses, PR1 , was found to be enhanced in crwn1crwn2 in a previous study [21] . The GO analysis showed that genes responsive to biotic and abiotic stimuli were predominantly up- and downregulated in crwn1crwn4 , consistent with the results of a previous study showing that CRWNs regulate genes related to immune responses [21] , [43] . The GO data implied that CRWNs are involved in many environmental stress responses. Plant material and growth conditions Arabidopsis thaliana Columbia-0 was used as the wild type. The mutants crwn1 to crwn4 , crwn1crwn4 , and crwn2crwn3 were described as linc1 to linc4 , linc1linc4 , and linc2linc3 disruptants, respectively, in a previous study [18] . The crwn1crwn2 mutants were made by crossing crwn1 and crwn2 . A. thaliana seeds were sterilized with sodium hypochlorite, vernalized at 4 °C for 1 day, and grown on ½ MS medium at 22 °C under a 16-h light/8-h dark photoperiod. The copper concentration in ½ MS medium was adjusted by adding copper (II) sulfate solution. Plasmid construction To create the CRWN-expressing lines, DNA fragments including the CRWN genomic DNA sequences and 2 kbp upstream from the start codon were cloned into the pENTR1A entry vector (Invitrogen, Carlsbad, CA, USA). pCRWN1 ::CRWN1-EYFP and pCRWN2 ::CRWN2-EYFP were constructed using the pGWB540 binary vector and pCRWN3 ::CRWN3-sGFP was constructed using the pMM1 binary vector [44] . The vectors were introduced into each of the crwn1–3 mutants by Agrobacterium tumefaciens -mediated transformation, and pCRWN1 ::CRWN1-GUS, pCRWN2 ::CRWN2-GUS, pCRWN3 ::CRWN3-GUS, and pCRWN4 ::CRWN4-GUS were each cloned into pGWB533 and introduced into WT. For the Co-IP assay, p35S ::CRWN1–4-GFP were previously described [18] and p35S ::CRWN1–3-tagRFP were each cloned into the pGWB560 binary vector. p35S ::CRWN4-tagRFP was constructed using the pSY1R binary vector in which GFP in the pSY1 binary vector is replaced with tagRFP [18] . To create lines overexpressing CA genes, the coding sequences of CA5 to CA10 were each cloned into the pENTER D-TOPO vector. p35S :: CA5 to p35S :: CA10 were constructed using the pGWB502 binary vector and introduced into crwn1crwn4 . As a positive control, pCRWN1 ::CRWN1-EYFP was also introduced into crwn1crwn4 . The sequences of the primers used in these experiments are shown in Supplementary Data 1 . Bright-field and fluorescence microscopy To visualize the subcellular localization of CRWNs, plants were stained with propidium iodide (10 μg/ml; Molecular Probes, Eugene, OR, USA) for 5 min. Confocal fluorescence images were obtained using a confocal laser scanning microscope (FV1200; Olympus, Tokyo, Japan) equipped with 405, 473, and 559 nm LD laser lines and a 100 × 1.40 N.A. oil immersion objective (UPlanSApo; Olympus), a 60 × 1.40 N.A. oil immersion objective (PlanApo; Olympus), a 40 × 1.30 N.A. oil immersion objective (UPlanFL; Olympus), and a 20 × 0.75 dry objective (UPlanSApo; Olympus). pCRWN1 ::CRWN1-GUS, pCRWN2 ::CRWN2-GUS, pCRWN3 ::CRWN3-GUS, and pCRWN4 ::CRWN4-GUS were fixed with 90% acetone on ice for 15 min. The fixed samples were washed with reaction buffer (50 mM phosphate buffer (pH 7.2), 2 mM K 3 Fe(CN) 6 , 2 mM K 4 Fe(CN) 6 , 0.1% NP-40) and were treated with 0.5 mM 5-bromo-4-chloro-3-indolyl-beta-D-glucuronide (X-Gluc) in reaction buffer at 37 °C for 16 h. After post fixation with 1% glutaraldehyde in reaction buffer for 2 h, the samples were treated with ethanol series (30, 50, 70, 90, 100%). Bright-field and fluorescence images were obtained using a BX51 microscope (Olympus). Image analysis was performed using ImageJ 1.51 g software (NIH, Bethesda, MD, USA). Immunoelectron microscopy Immunoelectron microscopy was performed as described in a previous study [45] with some modifications. Arabidopsis root tips were frozen in a high-pressure freezing machine (EM PACT; Leica Microsystems, Wetzlar, Germany). The samples were freeze-substituted with 0.25% glutaraldehyde and 0.1% uranyl acetate in 100% acetone at −80 °C for 4 days, and then gradually warmed (EM AFS; Leica Microsystems). The samples were washed with 100% acetone, infiltrated with methanol, and then embedded in LR White resin (London Resin Company Ltd., London, UK). Ultrathin sections (70–80 nm) on formvar-coated nickel grids were labeled with anti-GFP antibody (1:50, A11122; Thermo Fisher Scientific, Waltham, MA, USA) in 50 mM Tris-buffered saline (TBS). After washing with TBS, sections were labeled with 12-nm colloidal gold particles coupled to goat anti-rabbit IgG (1:20, AB_2338016; Jackson ImmunoResearch, West Grove, PA, USA). The sections were stained with 4% uranyl acetate for 20 min and then examined under a transmission electron microscope (JEM-1400; JEOL, Tokyo, Japan) at 80 kV. Immunofluorescence staining Seven-day-old seedlings expressing pCRWN1 ::CRWN1-EYFP, pCRWN2 ::CRWN2-EYFP, pCRWN3 ::CRWN3-sGFP, and p35S ::sGFP were fixed with 4% formaldehyde in phosphate-buffered saline (PBS) at 25 °C for 60 min and washed with PBS twice. After wiping the moisture off the samples, seedlings were chopped in chopping buffer (15 mM Tris–HCl pH 7.5, 2 mM EDTA, 0.5 mM spermine-4HCl, 80 mM KCl, 20 mM NaCl, and 0.1% Triton X-100) with a razor blade on a glass slide. The chopped sample was suspended in four volumes of nuclei suspension buffer (100 mM Tris–HCl pH 7.5, 50 mM KCl, 2 mM MgCl 2 , 5% sucrose, and 0.05% Tween-20) and then the solution was filtered through a 30-µm nylon mesh. A drop of the solution was placed on a cover slip and then allowed to dry overnight. After washing with 0.5% Triton X-100 in PBS, the nuclei were treated with 4% bovine serum albumin (BSA) in PBS at 25 °C for 30 min. The nuclei were then treated with anti-GFP antibody at 1:3000 (ab290; Abcam, Cambridge, UK) and 4 °C for 16 h. After washing with PBSt (0.05% Tween-20 in PBS) and blocking with 4% BSA in PBS, the nuclei were incubated with Alexa Fluor 488-conjugated anti-rabbit antibody at 1:1000 (A21206; Thermo Fisher Scientific) and 25 °C for 1 h. After washing with PBSt and pure water, the nuclei were mounted with VECTASHIELD Mounting Medium (H-1000; Vector Laboratories, Burlingame, CA, USA) and observed by a confocal microscope. Super-resolution microscopy The nuclei isolated from the plants expressing pCRWN1 ::CRWN1-EYFP, pCRWN2 ::CRWN2-EYFP, pCRWN3 ::CRWN3-sGFP, and p35S ::sGFP were placed on a cover slip and immunostained using anti-GFP antibody (ab290; Abcam) at 1:3000 and Alexa Fluor 488-conjugated anti-rabbit antibody at 1:1000, as mentioned above. The nuclei were mounted with ProLong™ Glass Antifade Mountant (P36982; Thermo Fisher Scientific) and stored at 4 °C. Super-resolution images were obtained using a STED microscope (SP8-gSTED; Leica Microsystems, Mannheim, Germany) equipped with a white light laser, a 592 nm STED laser, and a 100 × 1.40 N.A. oil immersion objective (HC PL APO CS2). The excitation wavelength at 488 nm and fluorescent signal in the range of 495–585 nm were detected by a HyD detector with 1.5–9.0-ns time gating. Images were obtained with 4 × line averaging and 2 × frame accumulation. The pixel size was set to 14 nm per pixel. Image processing was performed by deconvolution software (Huygens Professional ver.18.10.0p8 64b; Scientific Volume Imaging) with the default conditions. Images were further processed using ImageJ 1.51 g. Co-immunoprecipitation assay Fluorescent protein-conjugated CRWNs were transiently expressed in Nicotiana benthamiana leaves by Agrobacterium infiltration. The leaves were sampled at 4 days after inoculation. Immunoprecipitation was performed with a µMACS GFP Isolation Kit (Miltenyi Biotec, Auburn, CA, USA). The leaves (1.0–2.0 g) were homogenized in µMACS lysis buffer (2.0–4.0 ml) containing Protease Inhibitor Cocktail Complete (Roche) and then the extracts were centrifuged at 10,000 × g for 10 min to obtain the soluble lysate. Anti-GFP antibody-conjugated magnetic beads were added to the lysate and the mixture was incubated at 4 °C for 30 min with gentle shaking. The GFP-conjugated proteins were isolated using a magnetic column, in accordance with the manufacturer’s instructions. The purified proteins were analyzed by western blotting using an anti-GFP antibody at 1:2000 (ab290; Abcam), an anti-tagRFP antibody at 1:500 (R10367; Thermo Fisher Scientific), and HRP conjugated anti-rabbit antibody at 1:10000 (458; MBL, Aichi, Japan) Yeast two-hybrid assay The coding sequences of CRWN1–4 were each cloned into pGADT7 and pGBKT7. Y2HGold Yeast strain (Takara Bio, Shiga, Japan) was transformed using Frozen-EZ Yeast Transformation II (Zymo Research, Irvine, CA, USA). Transformants were selected on SD/-Leu/-Trip medium. The protein interactions were analyzed on SD/-Leu/-Trp/-His medium. Fluorescence in situ hybridization Flower buds were sampled from 5- to 6-week-old plants and fixed in Farmer’s solution (acetic acid:ethanol, 1:3) for 1 h at 25 °C. Fixed buds were washed with 70% ethanol and then with distilled water for 5 min. The buds were treated with an enzyme solution (2% w/v cellulose Onozuka RS, 0.5% w/v pectolyase Y-23, 10 mM citrate buffer, pH 4.5) at 37 °C for 1 h. The buds were broken by pipetting and then filtered through a 100-µm nylon mesh. The filtered nuclear solution was centrifuged at 5000 × g for 1 min and the pellet was resuspended in Farmer’s solution. A drop of the nuclear solution was placed on a glass slide and allowed to dry. Then, FISH was performed as previously described [46] . A centromere probe was amplified by PCR and labeled by nick translation using DIG-Nick Translation Mix (Sigma-Aldrich, St. Louis, MO, USA). Hybridized probes were visualized using a rhodamine-conjugated anti-digoxigenin antibody (Sigma-Aldrich). The number, size, and fluorescence intensity of FISH signals were measured using ImageJ 1.51 g. A binary image was generated from the fluorescent image and “Analyze Particles” in ImageJ was used to determine the signal size. To measure the fluorescence intensity, one pericentromeric signal was clipped from the raw image and “Measure” was used to determine the signal intensity. Subsequently, the background was subtracted from the signal intensity. RNA sequencing Total RNA was extracted from 14-day-old seedlings using an RNeasy Plant Mini Kit (Qiagen, Hilden, Germany) and treated with DNase I. Then, RNA-seq libraries were constructed using the TruSeq RNA library prep kit v2. The libraries were sequenced using a Nextseq 500 sequencer (Illumina, San Diego, CA, USA). Six independent biological replicates were analyzed for each genotype. Sequenced reads were mapped onto cDNA sequences of TAIR10 using Bowtie with –all –best –strata settings. Normalization and DEG detection were performed using the R package TCC ver. 1.28.0 [47] . The criteria for DEGs were as follows: fold value > 1.5 or <0.667 and FDR < 0.05. The GO analysis was performed using the PANTHER (Released 20171205). Chromatin integration labeling method A ChIL assay was performed as described previously with some modifications [25] . Twenty to thirty 9-day-old seedlings expressing pCRWN1 ::CRWN1-EYFP and p35S ::GFP were fixed with fixation buffer (1% formaldehyde in PBS) for 30 min under a vacuum and then 2 M glycine was added (final concentration, 150 mM). After washing with PBS, the seedlings were drained on a paper towel and then chopped in 50 µl of chopping buffer with a razor blade on a glass slide. The chopped sample was suspended in four volumes of nuclei suspension buffer (100 mM Tris–HCl pH 7.5, 50 mM KCl, 2 mM MgCl 2 , 5% sucrose, and 0.05% Tween-20) and then the solution was filtered through a 30-µm nylon mesh. Drops of the solution were added to wells of a 96-well plate and allowed to dry for several hours. The plate was either used immediately or stored at −80 °C. After washing with PBS, the nuclei were treated with 0.5% Triton X-100 and then with Blocking One P (Nacalai Tesque, Kyoto, Japan) for 20 min at 25 °C. After washing, anti-GFP antibody (ab290; Abcam) diluted 1:3000 in 0.1x Blocking One P in PBS was added and the plate was incubated for 6 h at 25 °C. After washing, secondary antibody solution (2 µg/ml oligo-conjugated anti-rabbit antibody, 0.1x Blocking One P, and 0.5 M NaCl in PBS) was added and the plate was incubated at 4 °C for 16 h. The nuclei were washed with ice-cold PBS and then treated with 1.77 µg/ml Tn5 transposase in dialysis solution (0.1 M NaCl, 0.1 mM EDTA, 1 mM DTT, 0.1% Triton X-100, 10% glycerol, 50 mM HEPES-KOH, pH 7.2) and then 2 nM Tn5-MEDS-B oligo in dialysis solution was added. After washing with PBS and dialysis solution, the nuclei were treated with TAPS-DMF buffer (5 mM MgCl 2 , 10% DMF, 10 mM TAPS-NaOH, pH 8.5) at 37 °C for 1 h and then the supernatant was removed and 0.2% sodium dodecyl sulfate (SDS) was added. After washing with T4 DNA ligase reaction buffer, the nuclei were treated with fill-in solution [200 U T4 ligase (New England Biolabs, Ipswich, MA, USA), 1.5 U T4 DNA polymerase (New England Biolabs), and 0.1 mM dNTP mix in T4 DNA ligase reaction buffer] at 25 °C for 30 min and then 0.2% (w/v) SDS was added. After washing with PBS and T7 RNA polymerase buffer, the nuclei were treated with in vitro translation solution [1000 U T7 RNA polymerase (TRL-252; Toyobo, Osaka, Japan), 40 U RNase inhibitor (Toyobo), 2 mM rNTPs in T7 RNA polymerase buffer] at 37 °C for 16 h and then 7 U DNase I (Nippon Gene, Tokyo, Japan) was added. The synthesized RNA was purified using an RNeasy MinElute Cleanup Kit (Qiagen) and cDNA was synthesized from purified RNA using a Verso cDNA Synthesis Kit (Thermo Fisher). Chromatin immunoprecipitation A ChIP assay was performed as described previously [48] . One gram of 9-day-old seedlings was frozen with liquid nitrogen, ground into fine powder with mortar and pestle, cross-linked in the nuclei isolation buffer (1% formaldehyde, 0.6% Triton X-100, 14.4 mM 2-mercaptoethanol,) with 1 mM Pefabloc SC (Merck, Hamburg, Germany) and complete protease inhibitor cocktail (Merck). M220 focused ultrasonicators (Covaris, Woburn, MA, USA) and milliTUBE 1 ml AFA Fiber (Covaris) were used for sonication. Sonicated samples were incubated with the antibody at 4 °C for overnight. Anti-histone H3 (ab1791; Abcam), anti-H4ac (06-866; Merck), and anti-H3K27me3 (07-449; Merck) were used. The samples were incubated with Protein G Magnetic Dynabeads (Thermo Fisher Scientific) at 4 °C for 2 h and then washed with low-salt RIPA buffer (50 mM Tris ⋅ HCl, pH 7.8, 150 mM NaCl, 1 mM EDTA, 1% Triton X-100, 0.1% SDS, 0.1% Sodium deoxycholate and 1% Complete protease inhibitor (Roche)), twice with high-salt RIPA buffer (50 mM Tris ⋅ HCl, pH 7.8, 500 mM NaCl, 1 mM EDTA, 1% Triton X-100, 0.1% SDS, 0.1% Sodium deoxycholate and 1% Complete protease inhibitor (Roche)), with LNDET buffer (250 mM LiCl, 1% IGEPAL, 1% Sodium deoxycholate, 1 mM EDTA, 10 mM Tris–HCl pH 7.8), and with TE buffer. After the elution buffer (10 mM Tris–HCl pH 7.8, 0.3 M NaCl, 5 mM EDTA, 0.5% SDS) was added to the beads, the beads were incubated overnight at 65 °C. The lysis was treated with 200 ng/ml RNaseA at 37 °C for 30 min and then treated with 800 ng/ml Proteinase K and 400 ng/ml glycogen at 37 °C for 2 h. After phenol chloroform extraction and ethanol precipitation, the pellet was suspended in Buffer EB (Qiagen). Collected DNA was used for real time PCR. Padlock FISH Twenty to thirty 9-day-old seedlings were fixed with fixation buffer (4% formaldehyde, 10 mM Tris–HCl pH 7.5, 10 mM EDTA, and 100 mM NaCl) for 20 min under a vacuum and then 2 M glycine was added (final concentration, 150 mM). The seedlings were drained on a paper towel and then chopped in 50 µl of chopping buffer with a razor blade on a glass slide. The chopped sample was suspended in four volumes of nuclei suspension buffer and then the solution was filtered through a 30-µm nylon mesh. Drops of the solution were placed on a cover slip and allowed to dry overnight. The cover slips were either used immediately or stored at −20 °C. Padlock FISH was performed as previously described [27] with some modifications and performed in a 55-μl SecureSeal chamber (Grace Bio-Labs, Bend, OR). After washing with 0.2% Triton X-100 in PBS, the samples were treated with 0.5 U/μl Eco RI at 37 °C for 30 min. After washing twice with buffer A (100 mM Tris–HCl pH 7.5, 150 mM NaCl and 0.05% Tween-20), the samples were treated with 0.2 U/μl of Lambda exonuclease (New England Biolabs) in Lambda exonuclease reaction buffer containing 0.2 μg/μl BSA and 10% glycerol at 37 °C for 30 min. After washing twice with buffer A, the nuclei were incubated with 0.1 μΜ Padlock probe in 2x SSC containing 20% formamide and 0.5 μg/μl sonicated salmon sperm at 37 °C for 15 min. The slides were washed with buffer B (2x SSC, 0.05% Tween-20) and buffer A and then treated with 0.1 U/μl T4 ligase (New England Biolabs) in T4 DNA ligase reaction buffer supplemented with 250 mM NaCl, 0.2 μg/μl BSA, and 10% glycerol at 37 °C for 15 min. Slides were washed in buffer B at 37 °C for 5 min, rinsed in buffer A and dehydrated in a series of 70, 85 and 100% ethanol. The nuclei were treated with 1 U/μl phi29 DNA polymerase (Fermentas, Burlington, Canada) in phi29 DNA polymerase reaction buffer supplemented with 0.25 mM dNTPs, 0.2 μg/μl BSA and 10% glycerol at 37 °C for 1 h and then rinsed in buffer A. 250 nM fluorescence-labeled detection probe in a solution of 2x SSC and 20% formamide was added to the sample and incubated at 37 °C for 20 min. After washing five times with buffer A and three time with PBS, the samples were stained with 500 ng/ml 4′,6-diamidino-2-phenylindole (DAPI) for 20 min. After washing three time with water, samples were mounted in Prolong Gold antifade reagent (Thermo Fisher Scientific). The sequence of the padlock probe and detection probe are shown in Supplementary Data 1 . The distance from the nuclear edge to the CA gene locus was quantified using ImageJ 1.51 g. In the young plants used here, nuclei from WT and crwn1crwn4 were of comparable size (Supplementary Fig. 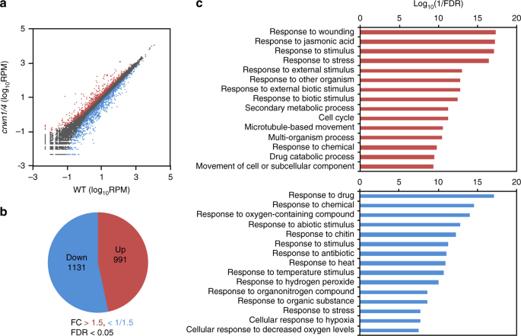Fig. 3: CRWNs affect gene expression pattern. aScatter plots of RNA-seq data comparing mRNA abundance between WT andcrwn1crwn4. Red marks denote mRNAs upregulated more than 1.5-fold (FDR < 0.05); blue marks denote those downregulated to <0.667-fold (FDR < 0.05); gray marks denote other mRNAs.bPie chart of differentially expressed genes (DEGs).cEnrichment analysis of GO terms for upregulated genes (top) and downregulated genes (bottom). GO analysis according to biological process. 9b ). 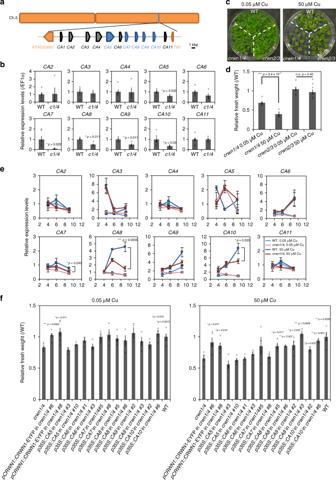Fig. 4: CRWNs elevate expression ofCAgenes. aSchematic figure of theCAgene locus on chromosome 5. Downregulated genes identified by qRT-PCR are shown in blue and otherCAgenes are shown in gray.bqRT-PCR analysis ofCAgenes in 2-week-old WT andcrwn1crwn4plants. Data were normalized to EF1α mRNA levels and are expressed as mean ± SEM relative to the WT value (defined as 1). Significance was determined using unpaired two-sidedt-test (n= 5 individual experiments). Each data point represents a cross mark.cWT,crwn1crwn4, andcrwn2crwn3grown under normal and excess copper conditions for 2 weeks.dFresh weight of 2-week-old WT,crwn1crwn4, andcrwn2crwn3grown under normal (n= 6 individual experiments) and excess copper conditions (n= 8 individual experiments). Fresh weights ofcrwn1crwn4andcrwn2crwn3were normalized against that of WT to calculate relative fresh weight and are expressed as mean ± SEM. Significance was determined using unpaired two-sidedt-test. Each data point represents a cross mark.eqRT-PCR analysis ofCAgene transcript levels in 4-, 6-, and 9-day-old WT andcrwn1crwn4under normal and excess copper conditions. Data were normalized to EF1α mRNA levels and are expressed as mean ± SEM relative to the value of 4-day-old WT under normal condition (defined as 1). Significance was determined using unpaired two-sidedt-test (n≥ 3 individual experiments).fFresh weight of 2-week-old WT,crwn1crwn4, andcrwn1crwn4expressing CRWN1-EYFP andCAgenes under normal and excess copper conditions. Fresh weights ofcrwn1crwn4andcrwn1crwn4expressing CRWN1-EYFP andCAgenes were normalized against that of WT to calculate relative fresh weight and are expressed as mean ± SEM. Significance was determined using unpaired two-sidedt-test (vscrwn1crwn4;n≥ 3 individual experiments). Each data point represents a cross mark. 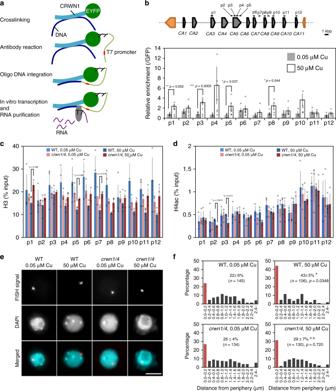Fig. 5: CRWNs regulate the position of theCAgene locus depending on copper concentration. aOutline of chromatin integration labeling (ChIL) method.bChIL-qPCR analyses using 12 primer pairs described as p1 to p12. Top image indicates the position of primer pairs at theCAgene locus. Data were normalized to ChILed DNA levels in GFP control and are expressed as mean ± SEM. Significance was determined using unpaired two-sidedt-test (n≥ 4 individual experiments). Each data point represents a cross mark.c,dChIP assay for histone H3 (c) and H4 acetylation (d) in theCAgene locus under normal and excess copper conditions. Data are expressed as mean ± SEM. Significance was determined using unpaired two-sidedt-test (n= 3 individual experiments). Each data point represents a cross mark.eVisualization of theCAgene locus in the nucleus by padlock FISH. In the merged panel, FISH signals are red and DAPI signals are cyan. Scale bar = 5 µm. Data are from single representative experiments that were reproduced three times.fThe distance between theCAgene locus and the nuclear edge was measured. The red bars in the histogram represent the nuclear periphery including the region 0.0 to 0.2 μm from the nuclear edge. The average percentage of theCAgene locus within the nuclear periphery with SEM from three independent replicates is shown. “n” represents the total number of FISH signals analyzed from all replicates. TheCAgene locus distribution data under normal conditions were compared with those under excess copper conditions in WT andcrwn1crwn4. Significance was determined using unpaired two-sidedt-test. Reporting summary Further information on research design is available in the Nature Research Reporting Summary linked to this article.